Reversed reactivity of anilines with alkynes in the rhodium-catalysed C–H activation/carbonylation tandem Development of multicatalytic approach consisting of two or more mechanistically distinct catalytic steps using a single-site catalyst for rapid and straightforward access of structurally complex molecules under eco-benign conditions has significance in contemporary science. We have developed herein a rhodium-catalysed C–H activation strategy which uses an unprotected anilines and an electron-deficient alkynes to C–C bonded products as a potential intermediate in contrast to the archetypical C–N bonded products with high levels of regioselectivity. This is followed by carbonylation of C–H bond activated intermediate and subsequent annulation into quinolines has been described. This rhodium-catalysed auto-tandem reaction operates under mild, environmentally benign conditions using water as the solvent and CO surrogates as the carbonyl source with the concomitant generation of hydrogen gas. The strategy may facilitate the development of new synthetic protocols for the efficient and sustainable production of chemicals in an atom-economic way from simple, abundant starting materials. New chemical approaches that enable rapid and straightforward access to synthetically important molecules by sequential transformations, which enhances the synthetic efficiency is one of the prime focuses in chemical science. Many enzymes are often capable of selectively processing a single substrate through a multiple sequential reactions and are often an inspiration for the development of new synthetic transformations [1] . Recently, ‘auto-tandem catalysis’, a strategy of association of two or more fundamentally different, that is, mechanistically distinct reactions promoted by a single-site catalyst, all of which occur under the same reaction conditions in a concurrent manner, is very attractive and highly desirable in organic synthesis [2] , [3] , [4] . In such tandem processes, potentially difficult work-up and product associated with the isolation and purification of the intermediates in multistep sequences can be avoided and the generation of chemical waste is also minimized. Development of such auto-tandem catalytic processes and a practically viable catalytic system is very challenging and sporadically mentioned due to the difficulty in the optimization of the separated processes independently [5] . More recent, transition-metal-catalysed C–H bond activation approach has provided a direct and an atom-economical synthetic strategy to achieve structurally complex molecules from simple, pre-functionalised substrates and this has implication in developing more efficient synthetic methodologies [6] , [7] , [8] , [9] , [10] , [11] . The pre-installed directing group assisted ortho -C–H activation has been explored by several research groups. In recent times, a rare examples of challenging meta -C–H activation using the template strategy is also reported [12] , [13] . However, transition-metal-catalysed direct oxidative coupling between simple arenes and activated alkenes via the non-directed C–H bond activation strategy (electrophilic metallation) is of great interest and reported by research groups of Fujiwara [14] , [15] , Glorious [16] , [17] , Yu [18] , [19] and others [20] , [21] . A gold-catalysed ethynylation of ‘deactivated’ arenes with electron-deficient alkynes is also documented [22] . Despite using pre-functionalised substrates for the C–H bond activation event, a regio- and stereoselectivity and use of excess arenes for improved reactivity towards transition metals are of potential concern. Hence, selective C–H functionalization of arenes through the non-directed C–H activation strategy is highly challenging and synthetically demanding. On the other hand, anilines serve as versatile precursors for the synthesis of N -heterocyclic scaffolds. In general, an aniline undergoes the Micheal-type 1,4-conjugate addition reaction with an electron-deficient alkyne and leads to usual carbon–nitrogen bonded product [23] . Transition-metal-catalysed hydroamination of alkynes (a formal addition of a N–H bond across a carbon–carbon multiple bond) for the synthesis of organo-nitrogen molecules is well documented ( Fig. 1a ) [24] , [25] . However, transition-metal-catalysed C–H bond activation of unprotected or ‘directing group-free’ amines is extremely rare [26] , [27] , [28] , [29] , [30] , [31] . Typically it proceeds via the formation of a five- or a six-membered metallacyclic intermediate and notably, in all such reports, either benzylic amines or ortho -aryl/vinyl anilines were used as the effective directing groups [26] , [27] , [28] , [29] , [30] . Recently, transition-metal-catalysed oxidative C–H activation/annulation of anilines with alkynes to indole derivatives using molecular oxygen as an oxidant is also reported ( Fig. 1b ) [32] , [33] . The reaction proceeded through either in situ formation of NH(OAc) or the Michael-type intermediate. However, to the best of our knowledge, there is no example of non-directed catalytic C–H bond activation of unprotected primary anilines [34] , [35] . 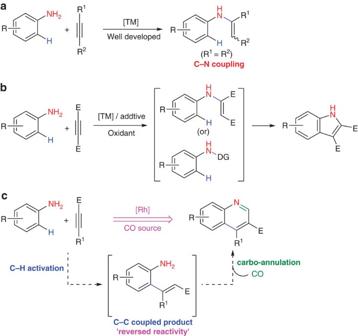Figure 1: Reactivity of unprotected anilines with alkynes. (a) Transition-metal-catalysed hydroamination of alkynes (a formal addition of a N–H bond across a carbon–carbon multiple bond). (b) Previous work involving transition-metal (TM)-catalysed oxidative C–H bond activation/annulation of anilines with alkynes to indole derivatives (DG, directing group; E, electron-withdrawing group). (c) In this report, reversed reactivity of anilines with alkynes in the rhodium-catalysed C–H activation/carbonylation tandem to quinoline derivatives. Figure 1: Reactivity of unprotected anilines with alkynes. ( a ) Transition-metal-catalysed hydroamination of alkynes (a formal addition of a N–H bond across a carbon–carbon multiple bond). ( b ) Previous work involving transition-metal (TM)-catalysed oxidative C–H bond activation/annulation of anilines with alkynes to indole derivatives (DG, directing group; E, electron-withdrawing group). ( c ) In this report, reversed reactivity of anilines with alkynes in the rhodium-catalysed C–H activation/carbonylation tandem to quinoline derivatives. Full size image Here we report a rhodium-catalysed C–H bond activation of unprotected (electron-rich primary) anilines with electron-deficient alkynes leading to formation of carbon–carbon bonded products as a potential intermediate in contrast to the archetypical carbon–nitrogen bonded products with high regio control. This is followed by carbonylation of C–H bond activated intermediate using CO surrogates and subsequent annulation reaction into the synthetically versatile 3-substituted quinolines is described ( Fig. 1c ). This rhodium-catalysed auto-tandem reaction operates under mild, environmentally benign conditions using water as a solvent and paraformaldehyde as a carbonyl source with the concomitant generation of hydrogen gas. Rhodium-catalysed C-H bond activation of anilines 3,4-(Methylenedioxy)aniline ( 1a ) and methyl propiolate ( 2a ) were selected as a benchmark substrates for the non-directed C–H bond activation strategy. Treatment of 3,4-(methylenedioxy)aniline 1a with methyl propiolate 2a in the presence of catalytic amount of rhodium catalyst resulted in 27% yield of C–H bond activated product, ethyl-3-(6-aminobenzo[ d ][1,3]dioxol-5-yl)acrylate ( 3a ) with the recovery of unreacted 1a in 49% ( Fig. 2a ). To gain more insight into this unobserved reactivity of anilines with alkynes, H/D exchange experiment was performed ( Fig. 2c ). When 3,4-(methylenedioxy)aniline ( 1a ) and p -toluidine ( 1a′ ) were separately treated with D 2 O in the presence of Rh(I)/dppm (1,1-bis(diphenylphosphino)methane) catalytic system, 77% of 1a was selectively deuterated to give [D]1a with high regio control ( Supplementary Figs 1 and 2 ) and whereas no H/D exchange was observed for 1a′ . These results imply that the carbon–carbon bond formation might begin with the ortho -C–H activation of 1a and can be proceeded via the electrophilic metalation (that is, non-directed strategy) [16] , [17] , [18] , [19] , [22] , and a resonance effect of substituents (+R group) is responsible for the regioselective C–H activation of anilines. 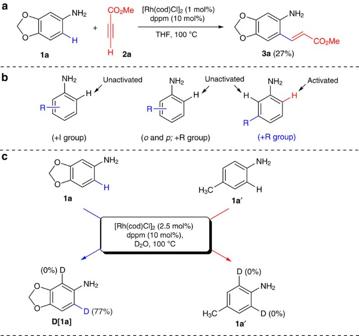Figure 2: Rhodium-catalysed C–H bond activation of unprotected anilines. (a) Rhodium-catalysed C–H bond activation of anilines with alkynes leading to the formation of carbon–carbon bonded product. (b) Effect of various substituents in the non-directed C–H bond activation of anilines. (c) Rhodium-catalysed regioselectiveortho-deuteration of anilines. Figure 2: Rhodium-catalysed C–H bond activation of unprotected anilines. ( a ) Rhodium-catalysed C–H bond activation of anilines with alkynes leading to the formation of carbon–carbon bonded product. ( b ) Effect of various substituents in the non-directed C–H bond activation of anilines. ( c ) Rhodium-catalysed regioselective ortho -deuteration of anilines. Full size image C-H bond activation/carbonylation tandem Recently, Gulías et al . [36] reported a rhodium-catalysed [5+1] cycloaddition of ortho -vinylphenols with carbon monoxide to lead a coumarin derivatives. Inspired by this result, we were encouraged to explore the possibility of utilization of the carbon–carbon bonded product ( ortho -vinylanilines) for further transformation. Thus, we planned to integrate rhodium-catalysed non-directed C–H activation strategy with the carbonylation reaction in an auto-tandem manner [37] . Development and scope After an extensive evaluation of combination of metal–ligand complexes, carbonyl sources, solvents and temperature ( Table 1 ; Supplementary Tables 1–6 ), we have optimized the finest reaction conditions for this auto-tandem catalysis. For example, the treatment of 3,4-(methylenedioxy)aniline ( 1a ) with methyl propiolate ( 2a , 1.1 equiv.) in the presence of catalytic amount of [Rh(cod)Cl] 2 :dppm (1:10 mol%) in tetrahydrofuran at 100 °C under 3 atm of CO for 12 h cleanly produced 4a in 49% yield with the recovery of the unreacted 1a in 42% ( Table 1 , entry 1). The reaction operates with double C–H bond activation under mild conditions with the formation of water as the by-product. To our delight, the same reaction was conducted using water as a solvent and yielded 4a in 46% ( Table 1 , entry 2) with the concomitant generation of hydrogen gas. The liberation of molecular hydrogen was qualitatively analysed by gas chromatography ( Supplementary Fig. 96 ). Table 1 Optimization of rhodium-catalysed C–H bond activation of anilines with alkynes and CO (surrogates). Full size table Interestingly, when aqueous formaldehyde was used as a carbon monoxide surrogate [38] , [39] , [40] in our auto-tandem approach, it showed a slight improvement in the product yield ( Table 1 , entry 3). Remarkably, excellent yields (up to 87%) were obtained when paraformaldehyde was used as a carbonyl source in CH 3 CN ( Table 1 , entry 6). Notably, addition of trace amount of water accelerated the reaction [41] and smoothly yielded the desired product ( Table 1 , entries 4–6). These results highlight the importance of water as a reaction medium, which may increase the solubility of paraformaldehyde and thus provide a slow release of CO gas available for the carbonylation reaction. Hence, water was used as an optimal solvent for this one-pot operation to afford a green synthetic protocol to the 3-substituted quinolines [42] (1 mol% of [Rh] yielded 3a in 93% and 2.5% mol% of [Rh] yielded 3a in 95%; entries 7–8). However, a three-component reaction of an aniline, an alkyne and an (aromatic) aldehyde to yield 2-substituted quinoline derivatives is a matured transformation in organic synthesis via typical Micheal-type 1,4-conjugate addition [42] , [43] . A multicomponent reaction of electron-deficient alkynes with amines and formaldehyde leads to polysubstituted pyrimidine derivatives were reported by Jiang and his co-workers and such type of product was not detected in our system [44] . It is very important to note that, in our reaction, paraformaldehyde and/or formalin solution were used as a carbonyl source (without using poisonous CO gas) and the reaction operates in an auto-tandem manner. The ‘auto-tandem’ catalysis consisting of a non-directed C–H bond activation of free anilines leads to C–C bonded intermediate, generation of carbon monoxide from CO surrogates, and carbonylation of C–H activated product followed by annulation reaction to yield 3-substituted quinolines with the generation of hydrogen gas. Indeed, there are no reports describing the direct syntheses of biologically important 3-substituted quinoline derivatives from simple, feedstock chemicals and usually accessed in a multistep synthetic procedures [45] . With the optimized reaction conditions in hand, we evaluated the substrate scope of the reaction with respect to the arene component and probed the generality of the auto-tandem process by generating a library of 3-substituted quinolines. As depicted in Fig. 3 , variety of electron-rich anilines was found to be the good commodity for this auto-tandem reaction. This is attributed to the electronic nature of the substituents (+R effect), and may facilitate the electrophilic metallation step much easier ( Fig. 2b ). Thus, a tool box of electron-rich anilines (alkoxy, crown-ether type, amide, alkyl, N -allyl and N -propargyl) were reacted smoothly with 2a via C–H bond activation and yielded the C–C coupled product as a potential intermediate (in contrast to the archetypical C–N bonded products) and followed by subsequent carbonylation using CO surrogates and annulation reaction to the 3-substituted quinolines in good to excellent yields (up to 95% isolated yield). The reaction is highly regio- and chemoselective and water and hydrogen gas is the only by-products. Remarkably, both allylic and propargylic groups were well tolerated under our reaction conditions. Alkyl substituted aniline ( 4j ) suffered from suppressed reactivity and observed poorer yield ( ∼ 6% by 1 H NMR). We presume this lower reactivity of aniline to be a consequence of decreased arene electron density: less η 2 coordination and more Lewis basic coordination to the metal centre. 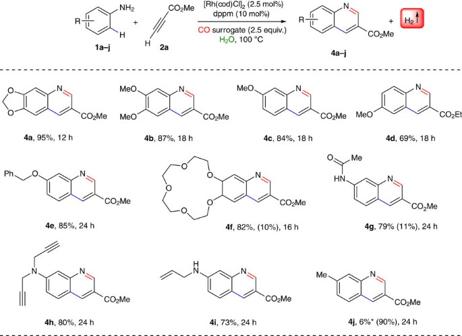Figure 3: Scope of anilines. Reaction conditions: anilines1a–j(0.25 mmol), methyl propiolate2a(0.275 mmol), [Rh(cod)Cl]2(2.5 mol%), dppm (10 mol%), (HCHO)n(2.5 equiv.) and 250 μl of H2O were heated at 100 °C under closed viol for specified time and depicted yields are isolated yields (yields in parentheses are recovery of the starting material). *Yield based on1H NMR of crude reaction mixture using toluene as an internal standard (using 1 mol% of the rhodium catalyst). Figure 3: Scope of anilines. Reaction conditions: anilines 1a–j (0.25 mmol), methyl propiolate 2a (0.275 mmol), [Rh(cod)Cl] 2 (2.5 mol%), dppm (10 mol%), (HCHO) n (2.5 equiv.) and 250 μl of H 2 O were heated at 100 °C under closed viol for specified time and depicted yields are isolated yields (yields in parentheses are recovery of the starting material). *Yield based on 1 H NMR of crude reaction mixture using toluene as an internal standard (using 1 mol% of the rhodium catalyst). Full size image Subsequently, we have also investigated the substrate scope with regard to the alkynes ( Fig. 4 ). Both carboxyl ester (entries 4k–4m ) and keto substituted ( 4n–4o ) terminal alkynes gave expected quinoline derivatives in excellent yields (up to 90% isolated yields). To our delight, dialkyl dicarboxylates smoothly underwent intermolecular annulation with aniline ( 1a ) and paraformaldehyde as a carbonyl source in water leading to the corresponding 3,4-disubstitutedquinoline derivatives ( 4p–4q) in good yields. Thus various electron-deficient alkynes including internal and terminal alkynylesters, linear and branched alkynylesters, and aryl ketoalkynes were shown good reactivity and yielded the desired 3- and 3,4-substituted quinolines in good to excellent yields with high regio- and chemioselectivity under mild, environmentally benign conditions with the liberation of molecular hydrogen. Importantly, in the reaction of 3,4-(methylenedioxy)aniline ( 1a ) with dimethyl acetylenedicarboxylate under standard reaction conditions with a shortened reaction time (6 h) yielded a mixture of the intermediate 3c (15%) and the desired product 4p with the yield of 13% ( Fig. 5 ). This result evidently proved that the auto-tandem approach proceeds through the C–C bonded intermediate. 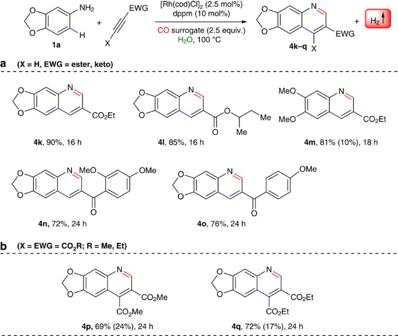Figure 4: Scope of alkynes. Reaction conditions: 0.25 mmol of 3,4-(methylenedioxy)aniline (1a) or 3,4-domethoxyaniline (1m), alkynes (0.275 mmol), [Rh(cod)Cl]2(2.5 mol%), dppm (10 mol%), (HCHO)n(2.5 equiv.) and 250 μl of H2O were heated at 100 °C under closed viol for specified time and depicted yields are isolated yields (yields in parentheses are recovery of the starting material). Figure 4: Scope of alkynes. Reaction conditions: 0.25 mmol of 3,4-(methylenedioxy)aniline ( 1a ) or 3,4-domethoxyaniline ( 1m ), alkynes (0.275 mmol), [Rh(cod)Cl] 2 (2.5 mol%), dppm (10 mol%), (HCHO) n (2.5 equiv.) and 250 μl of H 2 O were heated at 100 °C under closed viol for specified time and depicted yields are isolated yields (yields in parentheses are recovery of the starting material). 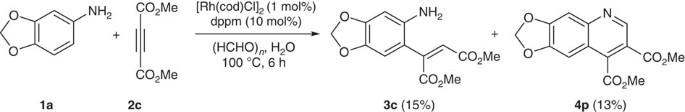Figure 5: Evidence for the formation of C–C bonded intermediate. Reaction of1awith DMAD (dimethyl acetylenedicarboxylate)2c. Full size image Figure 5: Evidence for the formation of C–C bonded intermediate. Reaction of 1a with DMAD (dimethyl acetylenedicarboxylate) 2c . Full size image We have also designed a three-step synthetic protocol for 6,7-dihydroxyquinoline-3-carboxamide ( 8 ), a tyrosine kinase inhibitors ( Fig. 6 ); which resulted in a 54% (overall) yield using our stragety [45] . 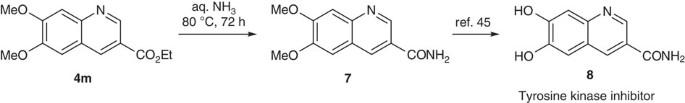Figure 6: Synthesis of8, a tyrosine kinase inhibitor. Reaction conditions: 0.25 mmol of4m(synthesized by our auto-tandem strategy) and 4 ml of aq. NH3were heated at 80 °C under closed viol for 72 h. Figure 6: Synthesis of 8 , a tyrosine kinase inhibitor. Reaction conditions: 0.25 mmol of 4m (synthesized by our auto-tandem strategy) and 4 ml of aq. NH 3 were heated at 80 °C under closed viol for 72 h. Full size image Carbonylation of ortho -vinylanilines using CO surrogates In addition to the one-pot operation, we speculated on the possibility where conditions could be developed to convert various ortho -vinylanilines to the corresponding quinoline derivatives via sequential carbonylation and intramolecular imination reactions using CO surrogates as the carbonyl source ( Fig. 7 ). However, performing carbonylation reactions both in industry and academia without the use of carbon monoxide (gasesous form, highly toxic, flammable and need of special high pressure equipment) is highly desired [39] , [40] , [46] . As described previously, we were hopeful with the Rh(I)/dppm catalytic system and CO surrogates in water as a carbonyl source to accomplish the carbonylation reaction of ortho -vinylanilines. This is followed by the trapping of aldehydic intermediate by the amine counterpart may lead to 3,4-disubstituted quinolines in one-pot operation. Alper et al . [47] reported Pd-catalysed oxidative cyclocarbonylation of ortho -vinylanilines to 2(1 H )-quinolinones. Indeed, as far as we know, carbonylation of ortho -vinylanilines using CO surrogates has never been reported. Thus, treatment of ( E )-2-(1,2-diphenylvinyl)-5-methoxyaniline, 5a (0.25 mmol) with paraformaldehyde (0.75 mmol) at 100 °C for 24 h with a catalytic amount of [Rh(cod)Cl] 2 (2.5 mol%) and dppm (10 mol%), using water as the solvent, resulted 7-methoxy-3,4-diphenylquinoline in 82% isolated yield ( 6a ) with the concomitant generation of hydrogen gas. Notably, the same reaction under 3 atm pressure of carbon monoxide yielded 6a in 16% (water as the only by-product). The reaction is general and a variety of ortho -vinylanilines were compatible with this transformation. Thus, electron-donating groups proceeded smoothly to provide the corresponding carboannulated products 6a–6b (up to 86% isolated yield), wherein electron-withdrawing groups ( p -NO 2 and m -CF 3 ) were found to be ineffective under standard conditions. This may be attributed to more Lewis basic coordination to the rhodium centre. However, it is noteworthy that halide substituents ( 5e–5f ) were well tolerated and yielded the desired products 6e–6f (80% of 6e and 79% of 6f , respectively), as this is advantageous for further synthetic elaborations with transition-metal catalysis thereby broadening the diversity of the products. 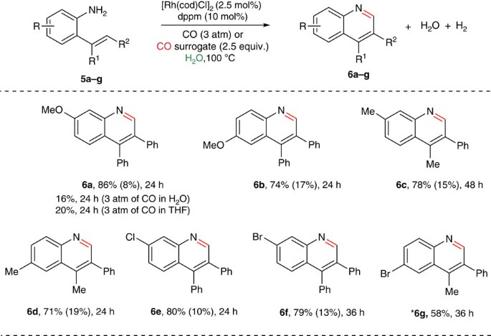Figure 7: Rhodium-catalysed carbonannulation ofortho-vinylanilines using CO (surrogate) in water. Reaction conditions:ortho-vinylanilines5a–g(0.25 mmol), [Rh(cod)Cl]2(2.5 mol%), dppm. (10 mol%), (HCHO)n(3 equiv.) and 250 μl of H2O were heated at 100 °C under closed viol for specified time and the yields in parenthesis are recovery of unreacted starting material. *Yields based on1H NMR of the reaction mixture (using 1 mol% of the rhodium catalyst). Figure 7: Rhodium-catalysed carbonannulation of ortho -vinylanilines using CO (surrogate) in water. Reaction conditions: ortho -vinylanilines 5a–g (0.25 mmol), [Rh(cod)Cl] 2 (2.5 mol%), dppm. (10 mol%), (HCHO) n (3 equiv.) and 250 μl of H 2 O were heated at 100 °C under closed viol for specified time and the yields in parenthesis are recovery of unreacted starting material. *Yields based on 1 H NMR of the reaction mixture (using 1 mol% of the rhodium catalyst). Full size image Mechanistic investigation To gain insight into the reaction mechanism, a series of control experiments, and deuterium-labelling studies were performed ( Fig. 8 ). 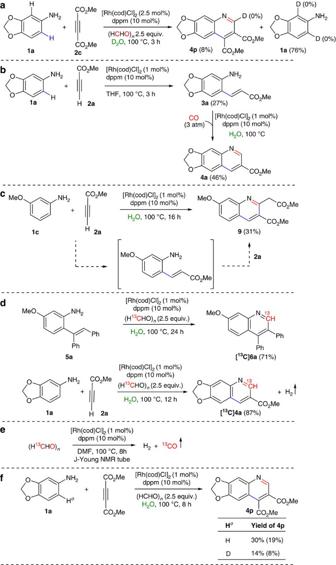Figure 8: Mechanistic investigation. (a) Irreversibility of regioselective C–H bond activation of1a. (b) Isolation of intermediates (C–C cross-coupled product) followed by carbonylation reaction. (c) Reaction of1cwith methyl propiolate (2a) in the absence of CO source. (d) Rhodium-catalysed auto-tandem reaction with labelled compounds. (e) Rhodium-catalysed CO formation from paraformaldehyde. (f) Kinetic isotopic experiments. (Yields in parentheses are isolated yields). Figure 8: Mechanistic investigation. ( a ) Irreversibility of regioselective C–H bond activation of 1a . ( b ) Isolation of intermediates (C–C cross-coupled product) followed by carbonylation reaction. ( c ) Reaction of 1c with methyl propiolate ( 2a ) in the absence of CO source. ( d ) Rhodium-catalysed auto-tandem reaction with labelled compounds. ( e ) Rhodium-catalysed CO formation from paraformaldehyde. ( f ) Kinetic isotopic experiments. (Yields in parentheses are isolated yields). Full size image Deuterium-labelling studies clearly confirmed the ortho -C( sp 2 )–H bond cleavage of the aniline is irreversible. Thus, the reaction of 1a with 2c using the standard reaction conditions in D 2 O was stopped before completion (3 h). Compounds 1a and 4p were isolated and their deuterium content was analysed by 1 H NMR. With both recovered compounds, no deuterium incorporation was observed suggesting that electrophilic metalation is irreversible in presence of 2c . However, it was observed that the cyclometalation of 1a is reversible in the absence of 2c ( Fig. 2c ). Under standard reaction conditions, the C–C bonded intermediate methyl-3-(6-aminobenzo[d][1,3]dioxol-5-yl)acrylate ( 3a ) was isolated in 27% from the reaction of 3,4-(methylenedioxy)aniline ( 1a ) with methyl propiolate 2a ( Fig. 8b ). Further, treatment of methyl-3-(6-aminobenzo[d][1,3]dioxol-5-yl)acrylate ( 3a ) with a catalytic amount of [Rh] under 3 atm of carbon monoxide cleanly produced 4a in 46% isolated yield. Notably, reaction of 3-methoxyaniline ( 1c ) and methyl propiolate 2a with a catalytic amount of [Rh] in the absence of carbonyl source with the prolonged time yielded, methyl 7-methoxy-2-(2-methoxy-2-oxoethyl)quinoline-3-carboxylate ( 8 ). This result strongly support that this auto-tandem catalysis is proceeding via the C–C bond formation ( Fig. 8c ; Supplementary Fig. 98 ). On the basis of the experimental details, other plausible pathways such as reaction via formation of –NHCHO, Michael addition intermediate, imine intermediate and [3,3] rearrangement have been discarded completely ( Supplementary Methods ). To understand the carbonylation process involving CO surrogates several labelling experiments were performed using 13 C-labelled paraformaldehyde. Indeed, labelling experiments unambiguously illustrated the formation of carbon monoxide from paraformaldehyde and therefore, utilized as a carbonyl source. Thus, under standard reaction conditions, using 13 C-paraformaldehyde as a carbonyl source both ortho -vinylaniline (( E )-2-(1,2-diphenylvinyl)-5-methoxyaniline ( 5a) and methyl-3-(6-aminobenzo[ d ][1,3]dioxol-5-yl)acrylate ( 3a ) ( in situ formation by the reaction of 3,4-(methylenedioxy)aniline, 1a with methyl propiolate, 2a ) predominantly yielded the corresponding 13 C-labelled quinoline derivatives ( Fig. 8d ). In addition, the reactivity of 13 C-paraformaldehyde in the presence of the rhodium catalyst under standard condition was investigated ( Fig. 8e ). Indeed, after 8 h, the formation of 13 C-labelled carbon monoxide and dihydrogen was qualitatively analysed on gas chromatography (GC) and GC–mass spectrometry (GC–MS) studies, and thus demonstrating the slow release of CO. However, in the presence of water as a reaction medium 13 CO 2 and H 2 were detected on GC and GC–MS ( Supplementary Figs 95 and 96 ). This is probably due to water–gas shift reaction [48] . On the basis of the above experimental findings and literature the precedent, we have proposed a plausible mechanism for the auto-tandem catalysis consisting of three mechanically distinct reactions, such as C–C cross-coupling via non-directed C–H activation, CO generation from CO surrogates and sequential carbonylation followed by annulation reaction catalysed by the single-site rhodium catalyst ( Fig. 9 ). The electrophilic metalation of aniline can provide the ortho -C–H bond activated product A ( Supplementary Fig. 97 ). Interaction of an alkyne with intermediate A can lead to intermediate B and subsequently alkyne insertion can lead to intermediate C . However, intermediate C can undergo proto-demetalation to provide the ortho -vinylaniline ( II ) in the absence of carbonyl source. Reaction of intermediate C with carbon monoxide ( in situ generated from CO surrogates) can lead to E via intermediate D . This is followed by the proto-demetalation of intermediate E and intramolecular imination to provide the expected quinoline moiety III . 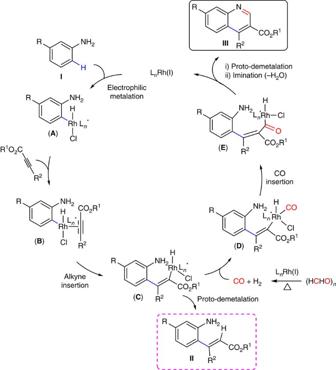Figure 9: Mechanistic rationale for the rhodium-catalysed auto-tandem construction of quinoline. Proposed catalytic cycles. Figure 9: Mechanistic rationale for the rhodium-catalysed auto-tandem construction of quinoline. Proposed catalytic cycles. Full size image Reversed reactivity of an aniline with an electron-deficient alkyne in the rhodium catalysis to lead to the formation of C–C coupled product as a potential intermediate in contrast to the archetypical C–N bonded products is disclosed. The product from this complementary approach (non-directed C–H activation strategy of free anilines) is integrated with sequential carbonylation and annulation reaction in an auto-tandem manner to lead to the 3-substituted quinolines with high rigio- and chemioselectivity is reported. This auto-tandem reaction operates under mild, environmentally benign conditions using water as a solvent and CO surrogates as a carbonyl source with extremely good atom-efficiency (only H 2 and H 2 O as by-products). Beyond the unique reactivity of this strategy, we anticipate that this auto-tandem catalysis will open a new avenue in the designing of new catalytic process for an efficient and a sustainable production of valuable targeted scaffolds from simple, feedstock chemicals in an atom-economic way. General procedure for this rhodium-catalysed auto-tandem reaction To a 10-ml clean, oven-dried screw cap reaction tube was added [Rh(cod)Cl] 2 (2.5 mol%), dppm 1,1-bis(diphenylphosphino)methane) (10 mol%), an aniline (0.25 mmol), CO surrogate (paraformaldehyde) (0.75 mmol), an alkyne (0.275 mmol) and water (250 μl) under argon atm. The reaction mixture was kept for heating at 100 °C for a specified time. After cooling to room temperature, reaction mixture was diluted with water (6 ml) and extracted with ethyl acetate (3 × 5 ml). The resultant organic layer was dried over anhydrous Na 2 SO 4 and the solvent was evaporated under reduced pressure. The crude mixture was purified by silica gel column chromatography (230–400 mesh size) using petroleum-ether/ethyl acetate as an eluting system. General procedure for rhodium-catalysed carbonylation of ortho -vinylanilines To a 10-ml clean, oven-dried screw cap reaction tube was added [Rh(cod)Cl] 2 (2.5 mol%), dppm (10 mol%), ortho -vinylaniline ( 5a–g ) (0.25 mmol), paraformaldehyde (0.75 mmol, 2.5 equiv.) and water (250 μl) under argon atm. The reaction mixture was heated at 100 °C for specified hours. After cooling at room temperature, reaction mixture was diluted with water (6 ml) and extracted with ethyl acetate (3 × 5 ml). The combined organic layer was dried over anhydrous Na 2 SO 4 and the solvent was evaporated. The crude product was purified by silica gel column chromatography (230–400 mesh size) using petroleum-ether/ethyl acetate as an eluent. All new compounds were fully characterized. For NMR and high-resolution mass spectrometry analysis in this article, see Supplementary Figs 3–93 . General information, materials, synthesis and characterization of compounds in this article ( D[1a] , 3a , 3c , 4a–4q , 6a–6g and 7–9 ), and experimental part for mechanistic investigations see Supplementary Methods . How to cite this article: Midya, S. P. et al . Reversed reactivity of anilines with alkynes in the rhodium-catalysed C–H activation/carbonylation tandem. Nat. Commun. 6:8591 doi: 10.1038/ncomms9591 (2015).